Interfacial Fe5C2-Cu catalysts toward low-pressure syngas conversion to long-chain alcohols Long-chain alcohols synthesis (LAS, C 5+ OH) from syngas provides a promising route for the conversion of coal/biomass/natural gas into high-value chemicals. Cu-Fe binary catalysts, with the merits of cost effectiveness and high CO conversion, have attracted considerable attention. Here we report a nano-construct of a Fe 5 C 2 -Cu interfacial catalyst derived from Cu 4 Fe 1 Mg 4 -layered double hydroxide (Cu 4 Fe 1 Mg 4 -LDH) precursor, i.e ., Fe 5 C 2 clusters (~2 nm) are immobilized onto the surface of Cu nanoparticles (~25 nm). The interfacial catalyst exhibits a CO conversion of 53.2%, a selectivity of 14.8 mol% and a space time yield of 0.101 g g cat −1 h −1 for long-chain alcohols, with a surprisingly benign reaction pressure of 1 MPa. This catalytic performance, to the best of our knowledge, is comparable to the optimal level of Cu-Fe catalysts operated at much higher pressure (normally above 3 MPa). Long-chain alcohols, containing more than five carbons, are key alternative fuels and feedstock to manufacture plasticizers, detergents, and lubricants [1] , [2] , [3] , [4] . Synthesis of long-chain alcohols (LAS) from syngas by a tandem strategy provides a facile, economical, and environment-friendly approach [5] , [6] , [7] . Among various binary catalyst systems (Cu–Fe [1] , [3] , [8] , Cu–Co [9] , [10] , Co–Mo [11] , [12] ), Cu–Fe binary candidates have attracted considerable attention in the production of long-chain alcohols. Previous studies on Cu–Fe binary catalysts show that a yield of long-chain alcohol as high as 0.014–0.144 g g cat −1 h −1 could be reached, albeit a relatively harsh reaction condition (3–8 MPa) is normally required. However, there is still room for the optimization of long-chain alcohols selectivity; more importantly, it is pivotal to develop catalyst system that works under mild reaction conditions [9] , [10] , [11] , [12] , [13] , [14] , [15] , [16] , [17] , [18] , [19] , [20] , [21] , [22] . Especially, the low pressure in practical operation gives a significant reduction in pressure drop, energy, and facility costs, which takes merits of both environmental and economic benefits [23] , [24] . To achieve this goal, a precise control over the type, dimension, and nature of Cu/Fe interface plays a key role in the production of LAS. Maintaining a high degree of Cu–Fe interface is decisive for shifting the products from hydrocarbons to long-chain alcohols. We have demonstrated previously that Fe 5 C 2 is very active for CO dissociation and C–C bond propagation, and thus is an excellent catalyst for the FTS reaction [25] , [26] , [27] . Lu et al. recently synthesized a 3DOM FeCu catalyst with atomic steps on the Cu surface involving planar defects and lattice strain, which showed excellent performance toward higher alcohols synthesis [3] , [16] . If we can prepare a highly dispersed iron carbide species over Cu, where CO is activated but not dissociated, it is possible to largely enhance the density of interfacial sites. This may render an optimized rate of C–C bond propagation on iron carbide sites and CO insertion on Cu/Fe 5 C 2 interfacial sites, and thus a high selective toward long-chain alcohols would be achieved. Layered double hydroxides (LDHs), with unique structure that metal cations are distributed in the hydroxide layers at an atomic level, have attracted extensive attention as catalyst precursors for higher alcohols synthesis [10] , [15] , [18] , [28] , [29] . In this report, we used Cu–Fe–LDHs as a precursor. After a structural topological transformation followed by an activation treatment [30] , [31] , [32] , [33] , [34] , Fe 5 C 2 cluster supported on Cu particle catalyst is obtained. Fe 5 C 2 clusters (~2 nm) are highly dispersed over the surface of Cu nanoparticles (~25 nm) which creates rich interfacial sites; and the Cu 4 Fe 1 catalyst with optimized Fe 5 C 2 –Cu interface exhibits a CO conversion of 53.2% and space time yield of 0.101 g g cat −1 h −1 for long-chain alcohols, at a low operation pressure (1 MPa). This is even comparable with the optimal space time yield level of other Cu–Fe binary catalysts at pressure of 3–8 MPa. Catalysts synthesis and characterizations The Cu x Fe y Mg 4 –LDH precursors with different Cu/Fe molar ratios (1/1, 2/1, 4/1, and 6/1, respectively) were prepared by a nucleation and aging separation method developed previously [15] . The XRD patterns (Fig. 1a ) show characteristic diffractions corresponding to an LDH phase (JCPDS 14-0281); SEM images display a typical plate-like hexagonal morphology (Supplementary Fig. 1 ). Actually, Cu 6 Fe 1 Mg 4 –LDH could hardly give an LDH phase due to the strong Jahn–Teller effect of Cu 2+ . The LDHs precursors were transformed to mixed metal oxides (MMO) that inherit the plate-like morphology (Supplementary Fig. 2 ) after thermal treatment. A CuO phase is predominant for these three samples (Fig. 1b ); while the diffractions at 35.8° and 37.1° confirm the formation of CuFe 2 O 4 spinel in XRD patterns. From HRTEM images (Supplementary Fig. 3 ), some nanoparticles uniformly embedded in the platelet matrix are clearly observed. The CuFe 2 O 4 nanoparticles are well-dispersed near CuO nanoparticles. According to the H 2 -TPR measurements (Fig. 1c ), the main peak shifts gradually from 280 °C to 350 °C with the increase of Cu/Fe ratio, which is ascribed to the enhanced amount of CuFe 2 O 4 spinel (a high reduction temperature) within CuO matrix (a low reduction temperature) [35] , [36] , [37] , as confirmed by XRD (Fig. 1b ) and HRTEM (Supplementary Fig. 3 ). The Cu 4 Fe 1 Mg 4 –MMO shows the strongest interaction between CuO and CuFe 2 O 4 species in accordance with HRTEM, possibly providing the most abundant and stable interfacial structure after activation. The precursors were reduced in syngas under optimized conditions to get the supported catalysts, which were denoted as Cu x Fe y ( x / y means the ratio between Cu and Fe). The Cu x Fe y catalysts show similar XRD patterns (Fig. 1d ) with metallic Cu. 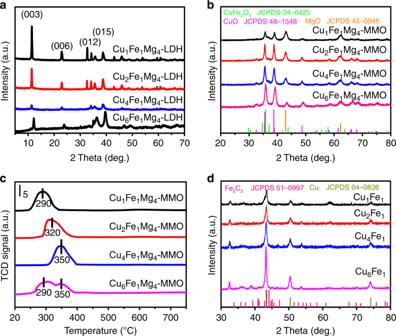Fig. 1: Catalysts characterizations. aXRD patterns of CuxFeyMg4–LDH precursors with three molar ratios of Cu/Fe (1:1, 2:1, 4:1, and 6:1, respectively).bXRD patterns of CuxFeyMg4–MMO calcined samples obtained from calcination of LDHs precursors.cH2-TPR profiles of CuxFeyMg4–MMO samples.dXRD patterns of CuxFeyobtained from activation of MMO samples in syngas (25% CO+25% H2+50% CO2) under optimum conditions (300 °C (2 h)+350 °C (1 h); rate: 2 °C min−1) and passivation. The average Cu particle sizes are 15.7, 18.4, 21.7, and 25.1 for Cu 1 Fe 1 , Cu 2 Fe 1 , Cu 4 Fe 1 , and Cu 6 Fe 1 samples, respectively (Supplementary Table 1 ). Moreover, no obvious diffraction of Fe crystalline is resolved, which indicates that Fe species is highly dispersed in the catalyst. Fig. 1: Catalysts characterizations. a XRD patterns of Cu x Fe y Mg 4 –LDH precursors with three molar ratios of Cu/Fe (1:1, 2:1, 4:1, and 6:1, respectively). b XRD patterns of Cu x Fe y Mg 4 –MMO calcined samples obtained from calcination of LDHs precursors. c H 2 -TPR profiles of Cu x Fe y Mg 4 –MMO samples. d XRD patterns of Cu x Fe y obtained from activation of MMO samples in syngas (25% CO+25% H 2 +50% CO 2 ) under optimum conditions (300 °C (2 h)+350 °C (1 h); rate: 2 °C min −1 ) and passivation. Full size image Catalytic results The catalysts were first evaluated under a relatively high pressure (3 MPa). 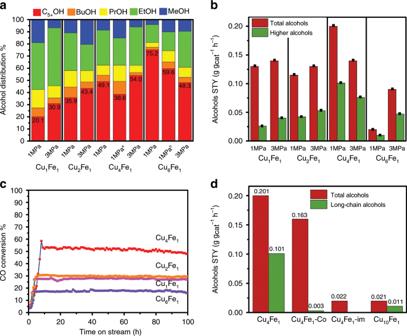Fig. 2: Catalytic performance. aAlcohol distribution normalized data to total alcohols selectivity (aWHSV = 4800 mL gcat−1h−1;bWHSV=1200 mL gcat−1h−1; C5+OH: long-chain alcohols, BuOH: butanol, PrOH: propanol, EtOH: ethanol and MeOH: methanol) andbalcohols STY at different pressures over catalysts with four Cu/Fe ratios (1/1, 2/1, 4/1, and 6/1) (reaction conditions: 27% CO+55% H2+18% N2; 260 °C; WHSV of 2400 mL gcat−1h−1).cTime-on-stream (TOS) evolution of CO conversion over the four catalysts within 100 h test at 1 MPa.dAlcohols STY of Cu4Fe1, Cu4Fe1-co, Cu4Fe1-im, and Cu10Fe1at 1 MPa. Figure 2a shows the alcohol distribution over catalysts with various activation treatments (Supplementary Tables 2 –6), from which both the activation atmosphere (syngas containing CO 2 ) and the two-stage activation procedure play a vital role in tuning the synergistic effect between Cu and Fe 5 C 2 . 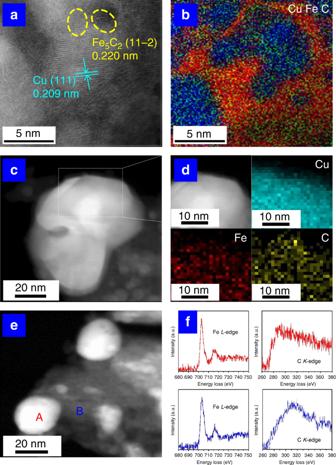Fig. 3: Structural studies on Cu4Fe1sample. aHRTEM image;bEELS mapping of Cu (blue), C (red), and Fe (green) of (a). quasi-in-situ STEM:cHAADF-STEM image;dEDS mapping of the selected region (white box inc) showing elemental distribution of Cu, C, and Fe;eHAADF-STEM image andfEELS curves of Fe L-edge and C K-edge selected from (e) (Spot A: red, Spot B: blue). 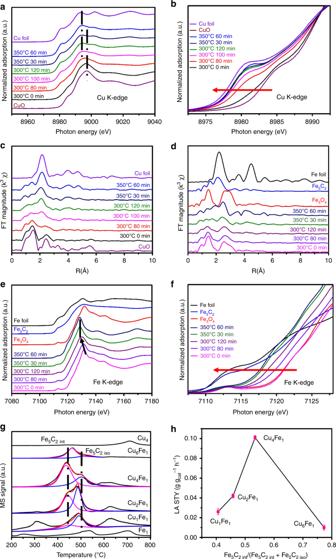Fig. 4: In situ XAS measurements of Cu4Fe1catalyst and CO-TPD measurements of Fe1, Cu4and CuxFeysamples. a,eIn situ XANES spectra at Cu K-edge and Fe K-edge of Cu4Fe1Mg4-MMO in syngas treatment to obtain Cu4Fe1catalyst (5% CO + 5% H2+ 10% CO2+ 80% He stream; 20 mL min−1) at different temperatures and time points, respectively.b,fEnlarged view of absorption edge selected from (a,e).c,dFourier transform magnitude of k3-weighted in situ Cu K-edge and Fe K-edge EXAFS spectra, respectively.gCO-TPD profiles of Fe1, Cu4, and CuxFeysamples.hLong-chain alcohols space time yield as a function of Fe5C2int/(Fe5C2int+ Fe5C2iso). Fe5C2int: interfacial Fe5C2; Fe5C2iso: isolated Fe5C2. The error bars are between 0.002 and 0.003. The sample activated in syngas containing CO 2 (Supplementary Table 4 ) could slow down the rate of reduction process and facilitate carburization of Fe to produce Fe 5 C 2 species, which would maintain the tiny size of Fe 5 C 2 to form abundant Cu–Fe 5 C 2 interfacial sites. The sample reduced in syngas shows diffraction peaks of both Cu and Fe 5 C 2 phase (Supplementary Fig. 4 ) and rather poor catalytic behavior for the production of LA, indicating less interfacial sites merged by poor dispersion of Fe 5 C 2 is not beneficial for the production of LA. The selectivity toward long-chain alcohols enhances gradually along with the increase of Cu/Fe ratio, reaching maximum at 54.0% for Cu 4 Fe 1 at 3 MPa (specific data in Supplementary Table 7 ). Cu 4 Fe 1 gives out the optimal space time yield (STY) (Supplementary Table 8 ) toward total alcohols (0.141 g g cat −1 h −1 ) and long-chain alcohols (0.076 g g cat −1 h −1 ) at 3 MPa. Fig. 2: Catalytic performance. a Alcohol distribution normalized data to total alcohols selectivity ( a WHSV = 4800 mL g cat −1 h −1 ; b WHSV=1200 mL g cat −1 h −1 ; C 5+ OH: long-chain alcohols, BuOH: butanol, PrOH: propanol, EtOH: ethanol and MeOH: methanol) and b alcohols STY at different pressures over catalysts with four Cu/Fe ratios (1/1, 2/1, 4/1, and 6/1) (reaction conditions: 27% CO+55% H 2 +18% N 2 ; 260 °C; WHSV of 2400 mL g cat −1 h −1 ). c Time-on-stream (TOS) evolution of CO conversion over the four catalysts within 100 h test at 1 MPa. d Alcohols STY of Cu 4 Fe 1 , Cu 4 Fe 1 -co, Cu 4 Fe 1 -im, and Cu 10 Fe 1 at 1 MPa. Full size image What attracts our attention most is the excellent long-chain alcohols production on Cu 4 Fe 1 under 1 MPa (Fig. 2 ; Supplementary Fig. 5 ). The Cu 4 Fe 1 has 38.6% at WHSV = 4800 mL g cat −1 h −1 with iso-conversion to other Cu x Fe y samples, although Cu 4 Fe 1 has higher value. The total alcohols yield (0.201 g g cat −1 h −1 ) of Cu 4 Fe 1 is much higher than hydrocarbons yield (0.111 g g cat −1 h −1 ), demonstrating the predominant production of alcohols rather than hydrocarbons (Supplementary Table 8 ). This means the high LA yield is the interplay of activity and selectivity. In addition, long-chain alcohols (C 5+ alcohols) give a higher yield than methanol (0.101 vs. 0.018 g g cat −1 h −1 ), which is among the highest level compared with previous work in Supplementary Table 9 . Normally, high reaction pressure (3–8 MPa) is required for long-chain alcohols synthesis; in this work, however, a low-pressure (1 MPa) syngas conversion to long-chain alcohols is attained. Significantly, Cu 4 Fe 1 catalyst at 1 MPa reaction condition shows a satisfactory stability: 5% decrease in activity is observed within a 100 h catalytic evaluation test (Fig. 2c ) and a satisfactory reproducibility (Supplementary Table 10 ). To understand the outstanding catalytic performance of Cu 4 Fe 1 , the impact of catalyst synthesis on its catalytic performance was investigated. Control samples with the same Cu/Fe ratio of 4/1 synthesized through conventional impregnation and co-precipitation methods were prepared (Supplementary Fig. 6 : termed as Cu 4 Fe 1 -im and Cu 4 Fe 1 -co, respectively), from which Cu–Fe 5 C 2 interfaces were rarely observed over those conventional catalysts. However, both catalysts produced scarcely any long-chain alcohols (Supplementary Table 11 ), indicating the unique interfacial structure derived from the LDHs synthesis route definitely changes the catalytic activity. Another two control samples of pure Cu (denoted as Cu 4 ) or pure Fe (denoted as Fe 1 ) were prepared based on a similar LDHs approach. The Cu 4 sample mainly shows methanol synthesis performance and the Fe 1 gives conventional FTS performance (Supplementary Table 11 ), in accordance with previous work [38] , [39] , [40] . When separate Cu 4 and Fe 1 catalysts were combined with various modes, long-chain alcohols could not be synthesized. This indicates that the Cu–Fe 5 C 2 synergistic effect is responsible for the production of long-chain alcohols. Therefore, the synergy of interfacial sites between Fe 5 C 2 and Cu is must for the long-chain alcohols (higher alcohols) synthesis from syngas. We performed further studies on samples with higher Cu/Fe molar ratios as 10:1 (termed as Cu 10 Fe 1 , Supplementary Fig. 7 ). Although both Cu 6 Fe 1 and Cu 10 Fe 1 samples have good selectivity of long-chain alcohols (Supplementary Table 12 ), the STY was low (Fig. 2b, d ), showing that a suitable Cu/Fe ratio is important for the best catalytic performance. This suggests that catalyst with rich Cu–Fe 5 C 2 interfaces derived from the LDHs precursor method could result in an excellent activity and selectivity toward long-chain alcohols even at a low reaction pressure. Fine structure characterizations To further understand the structural property of Cu x Fe y catalysts, the three samples (Cu 1 Fe 1 , Cu 2 Fe 1 , and Cu 4 Fe 1 ) were characterized by aberration-corrected scanning transmission electron microscopy (ac-STEM). For Cu 1 Fe 1 and Cu 2 Fe 1 samples (Supplementary Figs. 8 , 9 ), the lattice fringe of Cu (111) with 0.209 nm is clearly resolved; EDS mapping images of Cu, Fe, and C demonstrate the existence of Fe 5 C 2 nanoclusters on the surface of Cu nanoparticles. In the case of Cu 4 Fe 1 sample, Fig. 3a shows the lattice fringe of Cu (111) and Fe 5 C 2 (11-2); corresponding EELS mapping (Fig. 3b ) illustrates the modification of Cu by Fe 5 C 2 nanoclusters within a single Cu nanoparticle, which is also confirmed in another selected region in Supplementary Fig. 10 . Then, quasi-in-situ STEM measurements on the used catalyst after 1 MPa syngas conversion reaction were performed (Fig. 3 ). The EDX-mapping results (Fig. 3c, d ) also verified the homogeneous distribution of iron species on Cu. The phase of the iron species could be identified to be Fe 5 C 2 , as the catalyst shows sextets characteristics in Mössbauer spectrum (Supplementary Fig. 11 ) [16] , [41] . To further confirm the existence of iron carbide species on Cu particles, the electron energy-loss spectra (EELS) of C K-edge at the surface of Cu particle (Spot A) and support (Spot B) were studied (Fig. 3e, f ). For C K-edge spectra, Spot A displays a lower energy peak relative to Spot B, accompanied by a small peak at ~280 eV [42] , which again verifies the existence of carbide species on the surface of Cu particle. Fig. 3: Structural studies on Cu 4 Fe 1 sample. a HRTEM image; b EELS mapping of Cu (blue), C (red), and Fe (green) of ( a ). quasi-in-situ STEM: c HAADF-STEM image; d EDS mapping of the selected region (white box in c ) showing elemental distribution of Cu, C, and Fe; e HAADF-STEM image and f EELS curves of Fe L-edge and C K-edge selected from ( e ) (Spot A: red, Spot B: blue). Full size image In addition, in situ X-ray absorption near-edge structure (XANES) and extended X-ray absorption fine structure (EXAFS) experiments for Cu 4 Fe 1 Mg 4 –MMO at Cu K-edge and Fe K-edge (Fig. 4a, f ) were performed to reveal the structural change during the activation treatment process to obtain Cu 4 Fe 1 catalyst (in 20 mL min −1 5% CO+5% H 2 +10% CO 2 +80% He stream). The normalized Cu K-edge XANES spectra show a gradual decrease in the energy of absorption edge relative to CuO reference, accompanied with the appearance of edge features of metallic Cu, indicating a progressive reduction of CuO phase to metallic Cu. Corresponding fitting results (Supplementary Fig. 12 ) show that Cu species in Cu 4 Fe 1 is mainly metallic Cu with rather small amount of CuO x . Based on the results of previous reports [43] , [44] and observations in this work, Cu 0 is regarded as active site for CO adsorption/insertion. In the Cu K-edge EXAFS spectra, initially, the coordination environment of Cu 4 Fe 1 Mg 4 –MMO is consistent with CuO, in which the peaks at 1.5 Å and 2.5 Å are assigned to the first Cu–O coordination and Cu–Cu coordination, respectively [45] , [46] . During the activation process, the peak at 2.2 Å ascribed to Cu–Cu coordination shell gradually emerges and becomes predominant, further confirming the reduction to metallic Cu. In the case of Fe species, the normalized Fe K-edge XANES spectra show the reduction of CuFe 2 O 4 spinel to iron carbide phase along with the absorption edge moving to low energy. As shown in Fe K-edge EXAFS spectra, Fe–Fe coordination shell at 2.0 Å is observed at 350 °C, confirming the formation of iron carbide [3] , [47] , [48] . Based on above results, it is concluded that the new interfacial structure is well established from LDHs precursor through refined activation process. Fig. 4: In situ XAS measurements of Cu 4 Fe 1 catalyst and CO-TPD measurements of Fe 1 , Cu 4 and Cu x Fe y samples. a , e In situ XANES spectra at Cu K-edge and Fe K-edge of Cu 4 Fe 1 Mg 4 -MMO in syngas treatment to obtain Cu 4 Fe 1 catalyst (5% CO + 5% H 2 + 10% CO 2 + 80% He stream; 20 mL min −1 ) at different temperatures and time points, respectively. b , f Enlarged view of absorption edge selected from ( a , e ). c , d Fourier transform magnitude of k 3 -weighted in situ Cu K-edge and Fe K-edge EXAFS spectra, respectively. g CO-TPD profiles of Fe 1 , Cu 4 , and Cu x Fe y samples. h Long-chain alcohols space time yield as a function of Fe 5 C 2int /(Fe 5 C 2int + Fe 5 C 2iso ). Fe 5 C 2int : interfacial Fe 5 C 2 ; Fe 5 C 2iso : isolated Fe 5 C 2 . The error bars are between 0.002 and 0.003. Full size image Structure-performance relationship In addition, CO-TPD (Fig. 4g, h ) was performed to quantitatively study the amount of Fe 5 C 2 interfacial sites. As CO adsorption on Cu is rather weak and only be resolved through low-temperature TPD [49] , [50] , the observed desorption peaks are ascribed to iron species. In addition to the CO desorption from iron oxide at relatively low temperature (around 300 °C, for Cu 1 Fe 1 ) and reverse Boudouard reaction (above 600 °C), two desorption peaks at 440 °C and 490 °C (for Cu 1 Fe 1 , Cu 2 Fe 1 , Cu 4 Fe 1 , and Cu 6 Fe 1 ) could be attributed to CO desorption from iron carbide [51] , [52] . With Fe 1 as a reference, these two peaks (440 °C and 490 °C) are attributed to interfacial Fe 5 C 2 (Fe 5 C 2int ) and isolated Fe 5 C 2 (Fe 5 C 2iso ) species, respectively. Clearly, Cu 4 Fe 1 gives the largest integral peak area, indicating the most abundant total Fe 5 C 2 sites than other samples. We fitted and deconvoluted the two peaks to roughly estimate the ratio of Fe 5 C 2int /(Fe 5 C 2int +Fe 5 C 2iso ) for these four Cu x Fe y catalysts, and the results showed a volcanic correlation between the LA yield and the relative concentration of interfacial Fe 5 C 2 (Fig. 4h ). Cu 4 Fe 1 catalyst with a moderate Fe 5 C 2int ratio possesses the highest concentration of Fe 5 C 2 –Cu interface sites (Fe 5 C 2int ), accounting for the largest LA yield (0.101 g g cat −1 h −1 ). This demonstrates that the Fe 5 C 2 –Cu interfacial sites act as active center toward LA production. It is well-known that CO does not dissociate over Cu; while Fe 5 C 2 (or iron carbide in general) is beneficial for CO dissociation and subsequent C–C bond propagation [25] , [26] , [27] , [47] , [53] . The unique interfacial structure of ultrasmall Fe 5 C 2 clusters over Cu particles has conferred the Cu 4 Fe 1 catalyst a suitable construct for the production of long-chain alcohols production at syngas pressure as low as 1 MPa. De Jong et al. reported the size effect in supported iron carbides (2–7 nm) for Fischer–Tropsch reaction, in which a smaller particle size improved the coverage of CH x species (the monomer of carbon chain growth) [54] , [55] . In this work, long-chain alcohols synthesis at 1 MPa was achieved, which was described to the unique structure of Cu 4 Fe 1 catalyst. The Fe 5 C 2 nanoclusters, with an ultrasmall size (normally below 2 nm) on the surface of Cu nanoparticles, provide active sites for CO activation/dissociation and the resulting C–C bond propagation, which maintains the high activity of Cu 4 Fe 1 . As the reaction pressure decreases from 3 MPa to 1 MPa, hydrogen activation on catalyst surface is weakened (Supplementary Fig. 13 ), which reduces the rate of hydrogenation and hydrocarbons chain termination and thus enhances the growth of carbon chain. In contrast, the CO activation is promoted since CO molecule is prone to adsorb on a Cu-rich surface [56] , [57] . This facilitates the kinetic rate coordination between CO insertion and C–C coupling, and therefore significantly elevates the selectivity toward total alcohols and long-chain alcohols [58] , [59] , [60] . This is also verified by the α -ASF chain-lengthening probabilities analysis: the α -value for alcohols (0.72) at 1 MPa exceeds that for hydrocarbons (0.70), indicating the rate of CO insertion is larger than that of hydrocarbons chain termination (Supplementary Fig. 4 ). Therefore, a precise control over double-active-site in Cu 4 Fe 1 catalyst accounts for the high yield toward long-chain alcohols at 1 MPa. In summary, Cu 4 Fe 1 catalyst was synthesized from LDH precursor which exhibits a CO conversion of 53.2% and long-chain alcohols space time yield of 0.101 g g cat −1 h −1 , at a surprisingly benign pressure of 1 MPa. Combination of study verifies that highly dispersed Fe 5 C 2 nanoclusters are confined over the surface of Cu nanoparticles, forming abundant Fe 5 C 2 –Cu interfacial sites; and the synergistic interaction between Fe 5 C 2 clusters and Cu nanoparticle is responsible for the unique catalytic performance toward long-chain alcohol production at low pressure. This work not only discovers a catalyst with unique structure for LAS but also sheds light on the construct of binary metal catalyst. Catalysts synthesis The Cu x Fe y Mg 4 -LDH precursors with four Cu:Fe:Mg molar ratios of 1:1:4, 2:1:4, 4:1:4, and 6:1:4 (denoted as Cu 1 Fe 1 Mg 4 -LDH, Cu 2 Fe 1 Mg 4 -LDH, Cu 4 Fe 1 Mg 4 -LDH, and Cu 6 Fe 1 Mg 4 -LDH) were prepared by using a method of nucleation and aging separation developed in our laboratory [12] . Solution A was a mixture of Cu(NO 3 ) 2 ·3H 2 O, Fe(NO 3 ) 3 ·9H 2 O, and Mg(NO 3 ) 2 ·6H 2 O with various Cu:Fe:Mg molar ratios dissolved in 100 mL of deionized water ([Cu 2+ ] + [Mg 2+ ] + [Fe 3+ ] = 1.0 M). Solution B was obtained by dissolving NaOH and Na 2 CO 3 in the same volume of deionized water with [NaOH] = 1.6 M and [CO 3 2− ] = 2[Fe 3+ ]. Solution A and B were simultaneously added to a colloid mill rotating at 4000 rpm and mixed for 2 min. The resulting slurry was removed from the colloid mill and aged at 120 °C for 24 h. The final precipitate was filtered, washed thoroughly with deionized water, and dried at 60 °C for 24 h. General activation process: the Cu x Fe y Mg 4 -LDH precursors were calcined in air at 500 °C for 4 h at a heating rate of 2 °C min −1 to obtain mixed metal oxides (MMOs) (denoted as Cu 1 Fe 1 Mg 4 –MMO, Cu 2 Fe 1 Mg 4 –MMO, Cu 4 Fe 1 Mg 4 –MMO, and Cu 6 Fe 1 Mg 4 –MMO); subsequently, these MMOs materials were reduced in syngas atmosphere consisting of 25% CO+25% H 2 +50% CO 2 with a two-step-process—300 °C for 2 h and 350 °C for another 1 h at a heating rate of 2 °C min −1 (denoted as Cu 1 Fe 1 , Cu 2 Fe 1 , Cu 4 Fe 1 , and Cu 6 Fe 1 , respectively). In addition, based on Cu 4 Fe 1 Mg 4 -LDH precursor, the calcination temperature, activation procedure, and activation atmosphere were modulated to investigate their effects on catalytic performance, and the results were shown in Supplementary Tables 2 – 4 . Cu 4 , Fe 1 , and Cu 10 Fe 1 were prepared following above synthesis and activation process, which were derived from Cu 4 Al 1 Mg 4 –LDH, Fe 1 Mg 8 –LDH, and Cu 10 Fe 1 Mg 4 –LDH changing the ratio to Cu:Al:Mg = 4:1:4, Fe:Mg = 1:8, and Cu:Fe:Mg = 10:1:4, respectively (calcined samples: Cu 4 Al 1 Mg 4 –MMO, Fe 1 Mg 8 –MMO, and Cu 10 Fe 1 Mg 4 –MMO). Cu 4 Fe 1 -co as a reference sample was prepared by co-precipitated method [10] . A mixture of copper and iron nitrate (Cu/Fe molar ratio of 4/1) was precipitated with an aqueous solution of Na 2 CO 3 . After aging for 4 h, the precipitate was washed thoroughly with distilled water until pH = 7–8, and was dried at 60 °C for 12 h. Then, the sample was calcined and reduced via the same procedure described above. Cu 4 Fe 1 -im as a reference sample was prepared by incipient-wetness impregnation method [9] . In all, 8.0 g of CuO powdered sample was added into an aqueous solution containing 0.025 M iron nitrate. After impregnation for 4 h, the catalyst precursor was dried in air at 60 °C for 12 h followed by calcination and reduction in general activation process. Catalytic evaluation The catalytic evaluation was carried out in a 10 -mm fixed-bed stainless-steel reactor. In total, 1.0 g of MMO precursor was loaded on the catalyst bed, and the remaining volume of the reactor tube was filled with quartz beads of 20–40 mesh. Before reaction, the catalyst was activated in situ as mentioned above with a flow rate of 40 mL min −1 . After the reactor was cooled to room temperature, syngas with a flow rate of 40 mL min −1 (27% CO+55% H 2 +18% N 2 ) was introduced to purge the reaction line and reach the required pressure with nitrogen as an internal standard gas. The reaction was conducted at 260 °C. The outlet gas components (CO, H 2 , CH 4 , CO 2 , and N 2 ) after passing through a hot trap (180 °C) and a cold trap (5 °C) were determined using an online GC-2014C Shimadzu gas chromatograph with TCD detector (TDX-1 column) and FID detector (Al 2 O 3 packed column) using He as carrier gas. The liquid products were collected from the hot trap and cold trap, followed by determination offline with FID detector (RTX-5). 1,4-dioxane was used as internal standard for the aqueous products; and ethyl cyclohexane was used as an internal standard after extraction by cyclohexane. [ CO conversion was defined as:CO conversion( %);           = F_CO, in - F_CO, out/F_CO, in× 100 ]. (1) 
    Product selectivity was defined as:selectivity( mol%) = F_Ci× i/∑F_Ci× i× 100. (2) Where F is the moles of CO and product Ci (CO 2 , hydrocarbon, or alcohols) containing i carbon atoms. The mass balance and carbon balance have been calculated at each product and kept between 85 and 90%. The ASF chain growth probability α is calculated according to the equation: ln ( W n / n ) = n ln α + ln(1 − α ) 2 / α , where n is the number of carbon atoms in products; W n is the weight fraction of products containing n carbon atoms; and 1 − α is the probability of chain termination. Catalyst characterization Powder XRD measurements were performed on a Rigaku XRD-6000 diffractometer, using Cu Kα radiation ( λ = 0.15418 nm) at 40 kv and 30 mA, with a scanning rate of 5° min −1 and a 2 θ angle ranging from 3° to 90°. The phases of components were identified based on JCPDS standard cards. Scanning electron microscope (SEM; Zeiss SUPRA 55) with an accelerating voltage of 20 kV was performed. Aberration-corrected scanning transmission electron microscopy (ac-STEM), electron energy-loss spectroscopy (EELS), and element energy-dispersive spectroscopy (EDS) mapping measurements were carried out on a JEOL JEM-ARM200F instrument. The quasi-in-situ scanning transmission electron microscopy (STEM) and EDX-mapping measurements were performed on a FEI Tecnai G2 F20 microscope with an accelerating voltage of 120 kV. The sample was hold in glovebox in Ar atmosphere and transferred by a vacuum transfer TEM holder. The specific surface area determination and pore volume analysis were performed by Brunauer–Emmett–Teller (BET) and Barret–Joyner–Halenda (BJH) methods using a Quantachrome Autosorb-1C-VP Analyzer. Elemental analysis for Cu and Fe was performed using a Shimadzu ICPS-75000 inductively coupled plasma atomic emission spectrometer (ICP-AES). Hydrogen temperature-programmed reduction (H 2 -TPR) was measured on a Micromeritics ChemiSorb 2070 with a thermal conductivity detector (TCD). In a typical process, 100 mg of sample was sealed in a quartz tube reactor and pretreated in a Ar atmosphere at 150 °C for 2 h, followed by reduction in a stream of H 2 /Ar (1/9, v/v; a total flow rate of 40 mL min −1 ) at a heating rate of 10 °C min −1 up to 800 °C. Mössbauer spectrum experiments of the as-prepared catalysts were carried out at −268.8 °C. The spectrometer was calibrated using a standard α -Fe foil and was fitted with five sextets, which reflect Fe 5 C 2 and Fe 3 O 4 with different hyperfine parameters. The spectra components were identified according to their isomer shift, quadruple splitting, and magnetic hyperfine field. Magnetic hyperfine fields were calibrated with the 330 kOe field of α -Fe. In situ X-ray absorption fine structure spectroscopy (XAFS) at the Fe and Cu K-edge were acquired at 1W2 beamline of at Beijing Synchrotron Radiation Facility (BSRF) under transmission mode. The typical energy of the storage ring was 2.5 GeV with a maximum current of 250 mA. The Si (111) double-crystal monochromator was used. The powdered sample was first pressed into sheet and loaded into a reactor cell equipped with polyimide windows. The sample sheet was reduced in 5% CO+5% H 2 +10% CO 2 + 80% He stream with 20 mL min −1 , and underwent a heat treatment at 300 °C for 120 min then at 350 °C for 180 min (rate: 2 °C min −1 ). The XAFS spectra were collected 60 times h −1 in the whole process. All the collected spectra were processed and analyzed using Athena code within Ifeffit package. CO- or H 2 -temperature-programmed desorption (CO-TPD or H 2 -TPD) experiments were carried out in a fixed-bed reactor and detected by MS. 100 mg catalyst after reaction was exposed to CO or H 2 for 120 min in room temperature. The catalyst was switched to He exposure until the baseline of the CO or H 2 signal leveled off. Finally, the temperature was increased to 800 °C at 10 °C min −1 . The mass signal of 28 or 2 was monitored by quadruple mass spectrometer. The apparent kinetic order of H 2 was measured as follows: the catalytic test was performed at 260 °C with Cu 4 Fe 1 catalyst (0.1 g) in a gas flow rate of 40 mL min −1 in order to keep the H 2 conversion under 10%. For determining the order of H 2 , the partial pressure of H 2 was controlled from 22.5 to 45%.